Serotonin signals through a gut-liver axis to regulate hepatic steatosis Nonalcoholic fatty liver disease (NAFLD) is increasing in worldwide prevalence, closely tracking the obesity epidemic, but specific pharmaceutical treatments for NAFLD are lacking. Defining the key molecular pathways underlying the pathogenesis of NAFLD is essential for developing new drugs. Here we demonstrate that inhibition of gut-derived serotonin synthesis ameliorates hepatic steatosis through a reduction in liver serotonin receptor 2A (HTR2A) signaling. Local serotonin concentrations in the portal blood, which can directly travel to and affect the liver, are selectively increased by high-fat diet (HFD) feeding in mice. Both gut-specific Tph1 knockout mice and liver-specific Htr2a knockout mice are resistant to HFD-induced hepatic steatosis, without affecting systemic energy homeostasis. Moreover, selective HTR2A antagonist treatment prevents HFD-induced hepatic steatosis. Thus, the gut TPH1-liver HTR2A axis shows promise as a drug target to ameliorate NAFLD with minimal systemic metabolic effects. Nonalcoholic fatty liver disease (NAFLD) refers to a group of conditions characterized by excessive fat accumulation in the liver. It has become a serious public health problem globally, affecting more than half a billion people worldwide [1] , and is a leading cause of liver transplantation and hepatocellular carcinoma [2] , [3] . However, no pharmacological agents have been specifically approved for the treatment of NAFLD [4] , [5] , [6] , [7] . Therefore, it is necessary to better understand the mechanisms that contribute to the development of NAFLD. Serotonin (5-hydroxytryptamine (5-HT)) is a monoamine neurotransmitter that modulates central and peripheral functions. It is synthesized from the essential amino acid tryptophan and its production is regulated by the activity of tryptophan hydroxylase (TPH) and the availability of tryptophan [8] , [9] , [10] . The two distinct isoforms of TPH show mutually exclusive tissue expression patterns: TPH1 in peripheral non-neuronal tissues and TPH2 in neurons of the central and enteric nervous system [11] . Since 5-HT cannot cross the blood brain barrier, central and peripheral 5-HT systems are functionally separated [12] . Most of the peripheral 5-HT is synthesized by TPH1 in enterochromaffin cells of the gut. Once released to the blood circulation, the majority of 5-HT is taken up and sequestered into platelets, whereas the rest of 5-HT enters the systemic circulation and reaches peripheral tissues in free form [13] . Once entering systemic circulation, most of the free 5-HT is metabolized in liver and lung maintaining free 5-HT level in peripheral blood at very low levels [12] , [14] , [15] . 5-HT produced by TPH1 in gut and other peripheral tissues has been shown to exert specific biological effects dependent on the context of target tissues, e.g., adipose tissues, pancreatic β cells, bone, and liver [16] , [17] , [18] , [19] , [20] , [21] . While various functions of peripheral 5-HT are known, the direct role of 5-HT in regulating hepatic lipid metabolism in vivo is not well understood. Inhibiting peripheral 5-HT synthesis has been proposed to prevent NAFLD indirectly by protecting mice from obesity via thermogenesis in brown adipose tissue (BAT) [16] . Increased energy expenditure in BAT is thought to reduce hepatic lipid influx and thus prevent the development of NAFLD. In contrast, other studies demonstrated a direct effect of 5-HT on hepatic lipid accumulation in an in vitro model [22] . More recently, we have shown that short-term treatment of TPH inhibitors prevented the development of hepatic steatosis in mice fed a high carbohydrate diet without increasing energy expenditure in adipose tissues [23] . These data prompted us to further explore the detailed mechanism and function of 5-HT signals regarding liver energy metabolism in vivo. Here we show a novel role for gut-derived serotonin (GDS), through direct actions on liver, in the pathogenesis of hepatic steatosis. GDS regulates HFD-induced hepatic steatosis We first examined the expression of genes involved in 5-HT metabolism in order to evaluate whether liver could produce 5-HT. Unlike Slc6a4 , Maoa , and Maob , neither Tph1 nor Tph2 was expressed in the liver, suggesting that the hepatocyte can transport and metabolize 5-HT but is not likely to produce 5-HT (Fig. 1a ). Since nutrient infusion induces 5-HT production in the gut in human and the liver is the first organ to encounter GDS via the portal vein, free 5-HT levels in portal blood may reach concentrations sufficient to have endocrine effects on the liver [24] . To test this notion, we measured 5-HT levels in portal blood and peripheral blood of human subjects. Although the absolute levels of blood 5-HT varied among individuals, 5-HT concentrations were higher in portal blood relative to peripheral blood (Fig. 1b and Supplementary Fig. 1a, b ). Also, the ratio of 5-HT between portal and peripheral blood showed a tendency of positive correlation with markers associated with NAFLD such as blood levels of alanine transferase (ALT), gamma-glutamyltransferase (GTP), triglycerides (TG), and transient elastography controlled attenuation parameters (CAP) (Supplementary Fig. 1c ) [25] , [26] , [27] . Next, we assessed changes in 5-HT availability along the gut–liver axis on the liver in mice presenting with hepatic steatosis after 8 weeks of high-fat diet (HFD) feeding. Notably, HFD feeding increased both Tph1 expression and tissue 5-HT level in the gut, and free 5-HT levels in portal blood (Fig. 1c–e ). These data suggest that GDS production and portal 5-HT concentration can contribute to the development of NAFLD in both humans and mice. Fig. 1 Gut-derived 5-HT regulates HFD-induced hepatic steatosis. a mRNA expression of genes involved in 5-HT metabolism as assessed by RT-PCR in liver from 8-week-old C57BL/6J mice. b Plasma 5-HT concentrations of portal blood and peripheral blood in humans. Portal blood concentration set as 100%; n = 9 per group. c – e The 12-week-old male C57BL/6J mice were fed standard chow diet (SCD) or high-fat diet (HFD) for 8 weeks. c Tph1 mRNA expression in the duodenum, jejunum, ileum, and colon as assessed by qRT-PCR; n = 4 per group. d Duodenal 5-HT levels; n = 3 per group. e Plasma 5-HT levels in portal blood; n = 3 per group. f – h The 12-week-old WT and Tph1 GKO mice were fed SCD or HFD for 8 weeks. f Representative liver histology by hematoxylin and eosin (H&E) staining from HFD-fed WT and Tph1 GKO mice. Scale bars, 100 μm. g Nonalcoholic fatty liver disease activity score (NAS) of HFD-fed WT and Tph1 GKO mice; n = 7–10 per group. h Hepatic triglyceride levels; n = 6–10 per group. Data are expressed as the means ± SEM. * P < 0.5, ** P < 0.01, *** P < 0.001, Student’s t -test ( b – e , g ) or one-way ANOVA with post hoc Tukey’s test ( h ) Full size image In order to investigate the functional role of GDS in hepatic steatosis in vivo, we generated gut-specific Tph1 knockout (KO) ( Villin-Cre +/– ; Tph1 flox/flox , herein named Tph1 GKO) mice (Supplementary Fig. 1d, e ) and induced hepatic steatosis with 8 weeks of HFD feeding. Tph1 GKO mice showed no histological difference in liver compared to wild-type (WT) littermates ( Tph1 flox/flox ) in standard chow diet (SCD) feeding conditions (Supplementary Fig. 1f ). However, when hepatic steatosis was induced with 8 weeks of HFD feeding, hepatic lipid droplet accumulation, NAFLD activity score (NAS), and hepatic TG levels were dramatically reduced in the liver of HFD-fed Tph1 GKO mice (Fig. 1f–h ) [28] , indicating that reduced GDS production inhibits the progression of NAFLD. GDS does not affect systemic energy metabolism Hepatic steatosis develops when the rate of fatty acid (FA) input (influx and synthesis with subsequent esterification to TG) is greater than the rate of FA output (oxidation and outflux (very low-density lipoprotein (VLDL) secretion)) [29] . Previous studies reported that inhibition of peripheral 5-HT synthesis prevents obesity and metabolic dysfunction by increasing energy expenditure in BAT and beige adipocytes in inguinal white adipose tissue (iWAT) [16] , [17] . As such, we thoroughly examined the systemic metabolic phenotype of HFD-fed Tph1 GKO mice to evaluate whether increased energy expenditure improved hepatic steatosis indirectly by reducing FA influx in the liver. Upon HFD, Tph1 GKO mice, in comparison to WT littermates, showed no difference in body weight (BW) gain, glucose tolerance, insulin sensitivity, plasma lipid profiles, and adiposity (Fig. 2a–e , and Supplementary Fig. 1g ). BAT, iWAT, and epididymal white adipose tissue (eWAT) of Tph1 GKO mice showed no difference in organ weight and histology compared to WT littermates (Fig. 2f–k ). Especially, no obvious histological changes indicating BAT activation and beige adipogenesis were observed in BAT and iWAT of Tph1 GKO mice. In addition, neither Ucp1 expression in BAT and iWAT nor energy expenditure was different between Tph1 GKO mice and WT littermates (Fig. 2l–n ). These data indicate that GDS does not affect systemic energy metabolism in this context. Taken together, systemic energy metabolism does not seem to play a role in ameliorating HFD-induced hepatic steatosis in Tph1 GKO mice. Fig. 2 Gut-derived 5-HT does not affect systemic energy metabolism. a – n The 12-week-old WT and Tph1 GKO mice were fed SCD or HFD for 8 weeks. a Body weight trends; n = 6–10 per group. b Intraperitoneal glucose tolerance test (IPGTT) after 16 h fasting; n = 5 per group. c Intraperitoneal insulin tolerance test (IPITT) of HFD-fed WT and Tph1 GKO mice after 4 h fasting; n = 5 per group. d Plasma total cholesterol, free fatty acid, triglyceride, and high-density lipoprotein (HDL) cholesterol levels; n = 4–5 per group. e Percent fat body mass and lean body mass of HFD-fed WT and Tph1 GKO mice; n = 3 per group. f , h , j Adipose tissue to body weight ratio of BAT ( f ), iWAT ( h ), and eWAT ( j ); n = 6–10 per group. g , i , k Representative histology by H&E staining of sections from BAT ( g ), iWAT ( i ), and eWAT ( k ). Scale bars, 100 μm. l , m Relative mRNA expression of Ucp1 assessed by qRT-PCR in BAT ( l ) and iWAT ( m ) of HFD-fed WT or Tph1 GKO mice; n = 3 per group. n Metabolic parameters of HFD-fed WT or Tph1 GKO mice; n = 4 per group. Data are expressed as the means ± SEM. * P < 0.5, *** P < 0.001, Student’s t -test ( c , e , l , m ) or one-way ANOVA with post hoc Tukey’s test ( a , b , d , f, h , j , n ). VO 2 : oxygen consumption, VCO 2 : carbon dioxide production, RER: respiratory exchange ratio, XTOT: horizontal motor activity Full size image GDS regulates lipogenic pathways in the liver In order to identify the relevant metabolic pathways that prevent hepatic steatosis in Tph1 GKO mice, we performed gene expression analyses for an extensive array of metabolic markers. The expression of genes involved in lipogenesis were generally decreased in the liver of HFD-fed Tph1 GKO mice in comparison to WT littermates (Fig. 3a ). However, the expression of genes involved in FA uptake, FA oxidation, and VLDL secretion were not different between HFD-fed Tph1 GKO and WT littermates (Fig. 3b–d ). We next subjected Tph1 GKO and WT littermates to a methionine–choline-deficient (MCD) diet which induces hepatic steatosis by decreasing VLDL secretion rather than increasing FA input in the liver [30] . Liver histology, NAS, and hepatic TG concentrations of Tph1 GKO mice were not different in comparison to WT littermates fed an MCD diet (Fig. 3e–g ). As inhibition of GDS synthesis does not prevent hepatic steatosis in Tph1 GKO upon MCD diet, liver FA outflux is unlikely to mediate the GDS effects on liver. Taken together, inhibiting GDS synthesis ameliorates hepatic steatosis by downregulating lipogenic pathways in the liver. Fig. 3 Gut-derived 5-HT regulates lipogenic pathways in the liver. a – d The 12-week-old WT and Tph1 GKO mice were fed SCD or HFD for 8 weeks. Relative mRNA expression of genes involved in lipogenesis ( a ), FA uptake ( b ), FA oxidation ( c ), and VLDL secretion ( d ) as assessed by qRT-PCR in liver; n = 5 per group. e – g The 8-week-old WT and Tph1 GKO mice were fed MCD diet for 6 weeks. e Representative liver histology by H&E staining. Scale bars, 100 μm. f NAS; n = 3–4 per group. g Hepatic triglyceride levels; n = 3–4 per group. Data are expressed as the means ± SEM. ** P < 0.01, *** P < 0.001, Student’s t -test ( f , g ) or one-way ANOVA with post hoc Tukey’s test ( a – d ) Full size image HTR2A mediates the lipogenic action of GDS in the liver The physiological action of 5-HT is mediated through numerous 5-HT receptors (HTRs). To identify the HTR that mediates the role of GDS in the development of hepatic steatosis, we measured the expression of HTR genes in the liver (Supplementary Fig. 2a ). Interestingly, among the HTR genes found to be expressed at detectable levels in the liver, only Htr2a expression was markedly increased by HFD feeding (Fig. 4a ). To determine whether HTR2A mediates the steatotic effect of GDS in the liver, we generated mice harboring a floxed allele of Htr2a and crossed them with Albumin-Cre mice to generate liver-specific Htr2a KO ( Albumin-Cre +/– ; – Htr2a flox/flox , herein named Htr2a LKO) mice (Supplementary Fig. 2b, c ). Htr2a LKO mice showed slightly reduced liver size and weight compared with WT littermates ( Htr2a flox/flox ) after 8 weeks of HFD feeding (Fig. 4b, c ). Furthermore, HFD-fed Htr2a LKO mice showed decreased hepatic steatosis as examined by histology, NAS, and hepatic TG concentrations (Fig. 4d–f and Supplementary Fig. 2d ) without affecting BW, glucose tolerance, insulin sensitivity, and plasma lipid profiles (Supplementary Fig. 2e–h ). Similar to Tph1 GKO mice, the expression of genes involved in lipogenesis were decreased whereas genes involved in FA uptake, FA oxidation, and VLDL secretion were nearly the same in the liver of HFD-fed Htr2a LKO mice compared to WT littermates (Fig. 4g–j ). We also subject Htr2a LKO mice to an MCD diet for 6 weeks and found that liver histology, NAS, and hepatic TG levels were not different with MCD diet-fed WT littermates (Fig. 4k–m ). These results indicate that Htr2a LKO mice are protected against HFD-induced hepatic steatosis and is a phenocopy of Tph1 GKO mice in terms of hepatic steatosis. Fig. 4 HTR2A mediates the lipogenic action of GDS in the liver. a Relative mRNA expression of indicated HTRs as assessed by qRT-PCR in liver of SCD- and HFD-fed C57BL/6J mice; n = 4 per group. b – j The 12-week-old WT and Htr2a LKO mice were fed SCD or HFD for 8 weeks. Representative gross liver image ( b ) and liver weight ( c ) of HFD-fed WT and Htr2a LKO mice; n = 6–10 per group. Scale bar, 1 cm ( b ). d Representative liver histology by H&E staining from HFD-fed WT and Htr2a LKO mice. Scale bars, 100 μm. e NAS of HFD-fed WT and Htr2a LKO mice; n = 6–10 per group. f Hepatic triglyceride levels; n = 6–10 per group. g – j Relative mRNA expression of genes involved in lipogenesis ( g ), FA uptake ( h ), FA oxidation ( i ), and VLDL secretion ( j ) as assessed by qRT-PCR in liver; n = 5 per group. k – m The 8-week-old WT and Htr2a LKO mice were fed MCD diet for 6 weeks. k Representative liver histology by H&E staining. Scale bars, 100 μm. l NAS; n = 6–8 per group. m Hepatic triglyceride levels; n = 6–8 per group. Data are expressed as the means ± SEM. * P < 0.5, ** P < 0.01, *** P < 0.001, Student’s t -test ( a , c , e , l , m ) or one-way ANOVA with post hoc Tukey’s test ( f – j ) Full size image As HTR2B is the most highly expressed HTR in the liver and has been associated with hepatic carbohydrate metabolism [21] , we generated liver-specific Htr2b KO ( Albumin-Cre +/– ; Htr2b flox/flox , Htr2b LKO) mice and induced hepatic steatosis with 8 weeks of HFD feeding to examine the role of hepatic HTR2B in steatotic effects of GDS in the liver. HFD-fed Htr2b LKO mice showed no difference in liver histology, NAS, and hepatic TG levels compared with WT littermates ( Htr2b flox/flox ) (Supplementary Fig. 3a, b, c ). From these results, we confirmed that the protective effect against hepatic steatosis by reducing GDS production was highly specific for hepatic HTR2A. To further explore the molecular pathways underlying the decreased hepatic lipid accumulation in HFD-fed Htr2a LKO mice, we performed RNA-seq and profiled the liver transcriptomes of HFD-fed Htr2a LKO mice and WT littermates. We analyzed gene ontology (GO) gene sets by gene set enrichment analysis (GSEA). Among 5917 GO gene sets, 3614 gene sets with sufficient number of matched genes were analyzed and 617 gene sets and 27 gene sets were identified to be significantly enriched in WT littermates and Htr2a LKO mice, respectively (Supplementary Data file). Interestingly, gene sets which contribute to inflammation and fibrosis in nonalcoholic steatohepatitis pathogenesis as well as gene sets that contribute to steatosis were significantly less enriched in Htr2a LKO mice (Fig. 5a–c ) [31] , [32] , [33] , [34] , [35] , [36] , [37] , [38] , [39] , [40] . Quantitative reverse transcription polymerase chain reaction (qRT-PCR) analysis further confirmed that proinflammatory and profibrogenic genes were downregulated in the liver of HFD-fed Htr2a LKO mice (Fig. 5d ). These results suggest that inhibiting 5-HT signaling through hepatic HTR2A can inhibit the progression of NAFLD. Fig. 5 HTR2A mediates the inflammatory and fibrogenic action of GDS in the liver. a – d The 12-week-old WT and Htr2a LKO mice were fed HFD for 8 weeks. a – c GO gene sets were analyzed by GSEA for HFD-fed Htr2a LKO mice livers compared with WT littermates livers. Gene sets related to hepatic steatosis ( a ), inflammation ( b ), and fibrosis ( c ); n = 3 per group. d Relative mRNA expression of genes involved in inflammation and fibrosis as assessed by qRT-PCR in liver; n = 5 per group. Data are expressed as the means ± SEM. * P < 0.5, ** P < 0.01, *** P < 0.001, one-way ANOVA with post hoc Tukey’s test ( d ) Full size image HTR2A antagonist ameliorates HFD-induced hepatic steatosis Taken together with data from Tph1 GKO and Htr2a LKO mice, we have identified a previously unknown enterohepatic signaling pathway for hepatic steatosis mediated by GDS and hepatic HTR2A. These results led us to evaluate selective HTR2A antagonism as a novel therapeutic strategy for NAFLD. To this end, we tested sarpogrelate which is a selective HTR2A antagonist and mostly used as an antiplatelet agent for the treatment of peripheral arterial disease [41] , [42] , [43] , [44] . Mice were fed with HFD for 8 weeks and administered sarpogrelate daily using per os for the same period. As expected, sarpogrelate effectively decreased hepatic TG accumulation (Fig. 6a–c and Supplementary Fig. 4a ). In addition, closely resembling the effects of genetic deletion of Htr2a in the liver and Tph1 in the gut, sarpogrelate treatment resulted in decreased expression of genes involved in lipogenesis while genes involved in FA uptake, FA oxidation, and VLDL secretion were not changed in the liver (Fig. 6d–g ). We also examined the systemic metabolic effects of sarpogrelate since HTR2A is expressed in tissues outside the liver. Mice treated with sarpogrelate gained less BW upon HFD and their glucose tolerance was improved, while insulin tolerance was not affected (Supplementary Fig. 4b–d ). In addition, adipocyte size in iWAT and crown-like structure in eWAT were decreased in HFD-fed mice treated with sarpogrelate as compared to vehicle-treated HFD-fed mice (Supplementary Fig. 4e, f ). These results demonstrate that selective HTR2A antagonist can prevent hepatic steatosis in HFD-fed mice likely through common mechanisms shared with Tph1 GKO and Htr2a LKO mice. Fig. 6 HTR2A antagonist ameliorates HFD-induced hepatic steatosis. a – g The 12-week-old mice were fed SCD or HFD for 8 weeks and were treated with vehicle or sarpogrelate daily per os. a Representative liver histology by H&E staining from HFD-fed vehicle and sarpogrelate treated mice. Scale bars, 100 μm. b NAS of HFD-fed vehicle and sarpogrelate-treated mice; n = 6 per group. c Hepatic triglyceride levels; n = 5–6 per group. d – g Relative mRNA expression of genes involved in lipogenesis ( d ), FA uptake ( e ), FA oxidation ( f ), and VLDL secretion ( g ) as assessed by qRT-PCR in liver; n = 5 per group. Data are expressed as the means ± SEM. * P < 0.5, ** P < 0.01, *** P < 0.001, Student’s t -test ( b ) or one-way ANOVA with post hoc Tukey’s test ( c – g ) Full size image Peripheral 5-HT is emerging as a key regulator of systemic energy metabolism, modulating various physiological roles in multiple metabolic tissues [16] , [17] , [18] , [19] , [21] . Although 5-HT has been known to act on hepatocytes and promote lipid accumulation in vitro [22] , controversy still exists whether 5-HT acts directly on liver and regulates hepatic lipid metabolism in vivo. Here we demonstrate that inhibition of GDS synthesis by Tph1 GKO mice ameliorates hepatic steatosis independent of systemic energy homeostasis and Htr2a LKO mice revealed a phenocopy of Tph1 GKO mice. These results led us to propose GDS as a direct regulator of hepatic lipid metabolism via a gut–liver endocrine axis. In the present study, we have tested the effects of inhibiting GDS synthesis in two different hepatic steatosis models: HFD which increases fatty acid influx in the liver and MCD diet which reduces fatty acid outflux in the liver. Both Tph1 GKO and Htr2a LKO mice were effective only in HFD-induced liver steatosis without altering systemic energy homeostasis which suggest that blocking enterohepatic signaling pathways mediated by GDS and HTR2A represses TG accumulation in the liver. It is necessary to further identify detailed molecular mechanisms on how GDS regulates hepatic lipid disposal in the liver and how inhibition of HTR2A signaling reduces hepatic TG accumulation. Our findings also highlight the functional importance of hepatic HTR2A signaling in the progression of NAFLD. Inactivation of HTR2A signaling in the liver using Htr2a LKO attenuated hepatic steatosis independent of systemic energy homeostasis. Moreover, a selective HTR2A antagonist showed efficacy in improving hepatic steatosis as predicted by Tph1 GKO mice and Htr2a LKO mice phenotypes in HFD-induced hepatic steatosis. Thus, hepatic HTR2A is a potential target for therapies aiming to prevent the progression of NAFLD with minimal systemic metabolic effects. In addition, as the mortality increases geometrically with the increasing levels of fibrosis in NAFLD patients and many of genes involved in proinflammatory and profibrogenic pathways are downregulated in Htr2a LKO mice, it would be of interest to test whether HTR2A antagonism can effectively stop the progression of hepatic steatosis to fibrosis in the future [45] . A possible concern regarding the use of HTR2A antagonist for anti-NAFLD treatment is its potential adverse effects on hepatic regeneration after acute liver injury [20] . However, as sarpogrelate shows rare hepatotoxicity in real world practice, this concern might not be a problem to use it as an anti-NAFLD drug. Crane et al. [16] reported that HFD-fed Tph1 –/– mice indirectly improved NAFLD through UCP1-dependent thermogenic mechanisms. Oh et al. [17] demonstrated that, similar to Tph1 –/– mice, inhibition of 5-HT production in adipocytes had an anti-obesity effect by inducing thermogenesis in BAT and iWAT. In the present study, we demonstrated that HFD-fed Tph1 GKO mice are protected against hepatic steatosis without affecting systemic energy homeostasis. Taken together, our current model dictates that the metabolic phenotype of Tph1 –/– mice is the sum of the phenotype of Tph1 GKO mice and adipocyte-specific Tph1 KO mice. These findings suggest that there may be more various functions of 5-HT in different tissues. Thus, a more detailed study of the different roles of 5-HT using tissue-specific KO strategy will broaden our understanding of the function of this ancient neurotransmitter. Reagents d -Glucose, nonyl phenoxypolyethoxylethanol (NP-40), and sarpogrelate hydrochloride were purchased from Sigma-Aldrich (St Louis, MO, USA). TRIzol reagent was obtained from Invitrogen (Carlsbad, CA, USA). Animals and diets The Htr2a -targeted embryonic stem cell clone was obtained from the European Conditional Mouse Mutagenesis Program (EUCOMM) [46] . The mutant Htr2a allele (Htr2a tm1a(EUCOMM)Hmgu , Mouse Genome Informatics (MGI) [47] ID: 4946779, Supplementary Fig. 2b ) contains L1L2_Bact_P cassette located between exons 2 and 3 of the Htr2a gene, which is composed of a flippase recognition target (FRT) site followed by lacZ sequence and loxP site which is followed by human beta-actin promoter-driven neomycin resistance gene, SV40 polyA, a second FRT site, and second loxP site. A third loxP site is inserted downstream of exon 3 of the Htr2a gene. Targeted embryonic stem cells were injected into the blastocysts of BALB/c mice. C57BL/6N × BALB/c chimeric founders carrying the Htr2a tm1a(EUCOMM)Hmgu allele were crossed with C57BL/6J mice. The germ line transmissions of the F1 mice were analyzed and the confirmed offspring were crossed with transgenic flippase mice to remove the flanking FRT sites, resulting in Htr2a -floxed mice. Htr2a -floxed mice were backcrossed and maintained on a C57BL/6J genetic background. Primers for genotyping were as follows: forward primer 5′-TCTCAGACGTGGAAGGGTCT-3′ and reverse primer 5′-ACTGGTCACTGCTCAAAGGG-3′, which produce products of 252 base pairs (wild-type allele) or 320 bp ( Htr2a -floxed allele). To generate gut-specific Tph1 knockout ( Tph1 GKO) mice, Tph1 flox/flox (MGI: 3837399) mice were crossed with Villin-Cre (MGI: 2448639) mice. To generate liver-specific Htr2a knockout ( Htr2a LKO) and liver-specific Htr2b knockout ( Htr2b LKO) mice, Albumin-Cre (MGI: 2176228) mice were crossed with Htr2a flox/flox mice and Htr2b flox/flox (MGI: 3837400) mice. C57BL/6J mice were purchased from the Charles River Japan (Yokohama, Japan). Mice were housed in climate-controlled, specific pathogen-free barrier facilities under a 12  h light–dark cycle, and chow and water were provided ad libitum. Mice were fed SCD (Research Diet (New Brunswick, NJ, USA) D10001), HFD (Research Diet D12492, 60% fat calories), or MCD (Research Diet A02082002BR) diet. All animal experiments were complied with relevant ethical regulations. Experimental protocols for this study were approved by the institutional animal care and use committee at the Korea Advanced Institute of Science and Technology. Metabolic analysis To measure the metabolic rate, the mice were individually housed in an eight-chamber, open-circuit Oxymax/Comprehensive Lab Animal Monitoring System (Columbus Instruments, Columbus, OH, USA). After 1 day of acclimation, each mouse was assessed for oxygen consumption, carbon dioxide production, activity, and food intake for 72 h with access to diet and water ad libitum. Heat production was calculated as (3.815 + 1.232 × RER) × VO 2 , where RER (respiratory exchange ratio) was calculated as VCO 2 VO 2 –1 . Fat mass and lean body mass were measured using a Minispec time-domain nuclear magnetic resonance analyzer (Bruker Optics, Billerica, MA, USA). Glucose tolerance test and insulin tolerance test For the glucose tolerance test, 2 g kg −1 d -glucose in phosphate-buffered saline (PBS) was intraperitoneally injected into overnight-fasted mice. For the insulin tolerance test, 0.75 U kg −1 or 1 U kg −1 human insulin (Humulin R; Lilly, Indianapolis, IN, USA) was intraperitoneally injected into mice after fasting for 6 h. Blood samples were then obtained from the tail vein at 0, 15, 30, 45, 60, 90, and 120 min after injection. Glucose concentrations were measured using a Gluco DR Plus glucometer (Allmedicus, Anyang, Korea). Blood chemistry analysis Blood samples were collected by retro-orbital bleeding into plasma separation tubes with lithium heparin (BD Biosciences, Franklin Lakes, NJ, USA), followed by centrifugation at 1500 × g for 12 min at 4 °C. Enzymatic colorimetric assay kits for total cholesterol (Roche, Basel, Switzerland), high-density lipoprotein cholesterol (Roche), triglyceride (Roche), and free fatty acid (Wako, Osaka, Japan) were used to determine plasma levels on a Cobas 8000 modular analyzer (Roche) at GreenCross LabCell. Quantification of mouse serotonin To measure mouse platelet poor plasma (PPP) serotonin, blood samples were collected by retro-orbital bleeding or sampling from the portal vein. To acquire a PPP, we centrifuged twice to ensure no platelet contamination of supernatant; initially at 700 × g for 10 min and then 1792 × g for further 10 min. Quantification of serotonin was performed using an enzyme-linked immunosorbent assay kit (IBL International, Hamburg, Germany) according to the manufacturer’s instructions. To measure the levels of serotonin in the mouse gut, duodenum tissues were washed in PBS, followed by homogenization in RIPA buffer (Thermo Fisher Scientific, Waltham, MA, USA) using a FastPrep-24 (MP Biomedicals, Santa Ana, CA, USA). The homogenized tissues were centrifuged at 12,000 × g for 5 min at 4 °C. The supernatants were stored at −80 °C until analyses. Serotonin levels in tissue lysates were determined with an enzyme-linked immunosorbent assay kit (IBL International) or liquid chromatography-mass spectrometry method. Tissue serotonin levels were normalized to protein concentrations using a BCA Protein Assay Kit (Thermo Fisher Scientific) of homogenates. Quantification of hepatic triglyceride Liver tissues were homogenized in 5% NP-40 using FastPrep-24. To solubilize fat, the homogenates were heated to 95 °C for 5 min and cooled at 23 °C, and repeated. Triglyceride Reagent (Sigma-Aldrich) or PBS was added and incubated at 37 °C for 30 min to hydrolyze TG into glycerol. For the colorimetric assay of hydrolyzed TG levels, samples were incubated with Free Glycerol Reagent (Sigma-Aldrich) at 37 °C for 5 min. Differences in absorbance at 540 nm between hydrolyzed or non-hydrolyzed TG were quantified using a glycerol standard (Sigma-Aldrich). TG contents were normalized by the protein concentrations of homogenates, which were measured with a BCA Protein Assay Kit. Quantitative RT-PCR analysis Total RNA extractions from harvested tissues were performed using TRIzol according to the manufacturer’s protocol. After TURBO DNase (Invitrogen) treatment, 2 μg of total RNA was used to generate complementary DNA with Superscript III reverse transcriptase (Invitrogen). Quantitative RT-PCR was performed with Fast SYBR Green Master Mix (Applied Biosystems, Foster City, CA, USA) and a Viia 7 Real-time PCR System (Applied Biosystems) according to the manufacturer’s instructions. Gene expression was relatively quantified based on the delta delta Ct (threshold cycle) method with the beta-actin gene as a reference gene. 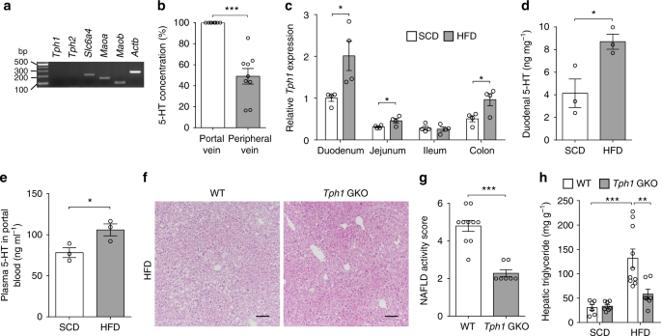Fig. 1 Gut-derived 5-HT regulates HFD-induced hepatic steatosis.amRNA expression of genes involved in 5-HT metabolism as assessed by RT-PCR in liver from 8-week-old C57BL/6J mice.bPlasma 5-HT concentrations of portal blood and peripheral blood in humans. Portal blood concentration set as 100%;n= 9 per group.c–eThe 12-week-old male C57BL/6J mice were fed standard chow diet (SCD) or high-fat diet (HFD) for 8 weeks.cTph1mRNA expression in the duodenum, jejunum, ileum, and colon as assessed by qRT-PCR;n= 4 per group.dDuodenal 5-HT levels;n= 3 per group.ePlasma 5-HT levels in portal blood;n= 3 per group.f–hThe 12-week-old WT andTph1GKO mice were fed SCD or HFD for 8 weeks.fRepresentative liver histology by hematoxylin and eosin (H&E) staining from HFD-fed WT andTph1GKO mice. Scale bars, 100 μm.gNonalcoholic fatty liver disease activity score (NAS) of HFD-fed WT andTph1GKO mice;n= 7–10 per group.hHepatic triglyceride levels;n= 6–10 per group. Data are expressed as the means ± SEM. *P< 0.5, **P< 0.01, ***P< 0.001, Student’st-test (b–e,g) or one-way ANOVA with post hoc Tukey’s test (h) The sequences of primers are given in Supplementary Table 1 . Histological analysis Mouse liver, inguinal white adipose tissue, epididymal white adipose tissue, and interscapular brown adipose tissue were harvested and fixed in 10% neutral buffered formalin solution (Sigma-Aldrich) and embedded in paraffin. The 5 μm-thick tissues sections were deparaffinized, rehydrated, and stained with hematoxylin and eosin (H&E). For quantitative evaluation of hepatic steatosis, NAS, which consists of steatosis, lobular inflammation, and ballooning, was used. NAS was determined by a single certified pathologist, blinded for other information. Quantification of human blood serotonin All experiments using human participant blood samples were complied with relevant ethical regulations. After previous approval by the institutional review board of Severance Hospital (4-2015-0184), and written, informed consent by all subjects, 9 living donors for liver transplantation were included in this study. Clinical data are given in Supplementary table 2 . Body weight and height were measured using a digital scale, and body mass index was calculated by dividing weight (kg) by the square of height (m 2 ). Laboratory parameters including complete blood count and differential count, calcium, phosphorus, glucose, blood urea nitrogen, creatinine (Cr), uric acid, cholesterol, total protein, albumin, alkaline phosphatase, aspartate transferase, ALT, total bilirubin, gamma-GTP, TG, high-density lipoprotein (HDL) cholesterol, low-density lipoprotein (LDL) cholesterol, sodium, potassium, chloride, prothrombin time, and activated prothrombin time were measured within 4 weeks before living donor hepatectomy. Transient elastography was performed using the liver Fibroscan (Echosens, Paris, France). Donor hepatectomy was performed according to standardized procedures. Blood samples for serotonin measurements were drawn simultaneously from the portal vein and peripheral veins during operation. Human PPP serotonin levels were measured using ClinRep high-performance liquid chromatography kit (Recipe, Munich, Germany) at GreenCross LabCell (Yongin, Korea). RNA-sequencing Total RNA was isolated using a RNeasy Plus Mini kit (QIAGEN) according to the manufacturer’s instructions. The integrity of the total RNA was assessed using an Agilent 2100 Bioanalyzer System (Agilent Technologies) and an Agilent RNA 6000 Nano Kit (Agilent Technologies). Samples with an RNA Integrity Number (RIN) value >8 were selected for use. Libraries were constructed using 1 μg total RNA. The RNA sequencing library was prepared using a TruSeq RNA Sample Prep kit (Illumina) and sequencing was performed using an Illumina NextSeq500 to generate 100 bp paired-end reads. FastQC (FastQC v0.11.3) and cut-adapt (v1.1) were used to filter out sequencing reads of low quality, and the retained reads were mapped to mouse genome build mm10 using TopHat (TopHat v2.0.11) with default parameters. HTseq (v0.9.1) was used to generate raw read counts. GSEA was performed using the GenePattern tool from the Broad Institute, with version of 5.2 of the Molecular Signature Database (MSigDB; http://www.broadinstitute.org/gsea/msigdb/index.jsp). HFD-fed Htr2a LKO mice ( n = 3) were compared with WT littermates ( n = 3), and representative significantly less enriched gene sets with nominal P value of less than 0.05 are presented. Statistics All values are expressed as the mean ± standard error of mean and analyses were performed using the SPSS Statistics version 23 (SPSS, Inc., Chicago, IL, USA). Two-tailed Student’s t -test or one-way analysis of variance (ANOVA) with post hoc Tukey’s test were used to compare groups. 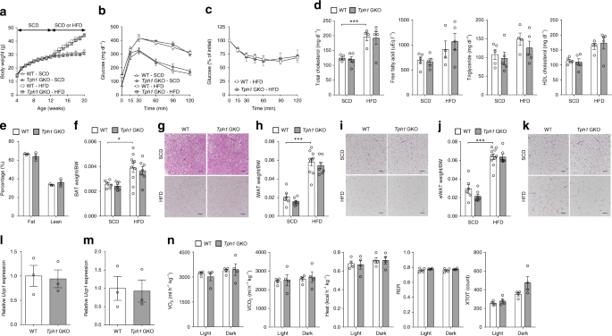Fig. 2 Gut-derived 5-HT does not affect systemic energy metabolism.a–nThe 12-week-old WT andTph1GKO mice were fed SCD or HFD for 8 weeks.aBody weight trends;n= 6–10 per group.bIntraperitoneal glucose tolerance test (IPGTT) after 16 h fasting;n= 5 per group.cIntraperitoneal insulin tolerance test (IPITT) of HFD-fed WT andTph1GKO mice after 4 h fasting;n= 5 per group.dPlasma total cholesterol, free fatty acid, triglyceride, and high-density lipoprotein (HDL) cholesterol levels;n= 4–5 per group.ePercent fat body mass and lean body mass of HFD-fed WT andTph1GKO mice;n= 3 per group.f,h,jAdipose tissue to body weight ratio of BAT (f), iWAT (h), and eWAT (j);n= 6–10 per group.g,i,kRepresentative histology by H&E staining of sections from BAT (g), iWAT (i), and eWAT (k). Scale bars, 100 μm.l,mRelative mRNA expression ofUcp1assessed by qRT-PCR in BAT (l) and iWAT (m) of HFD-fed WT orTph1GKO mice;n= 3 per group.nMetabolic parameters of HFD-fed WT orTph1GKO mice;n= 4 per group. Data are expressed as the means ± SEM. *P< 0.5, ***P< 0.001, Student’st-test (c,e,l,m) or one-way ANOVA with post hoc Tukey’s test (a,b,d,f, h,j,n). VO2: oxygen consumption, VCO2: carbon dioxide production, RER: respiratory exchange ratio, XTOT: horizontal motor activity P values below 0.05 were considered statistically significant. 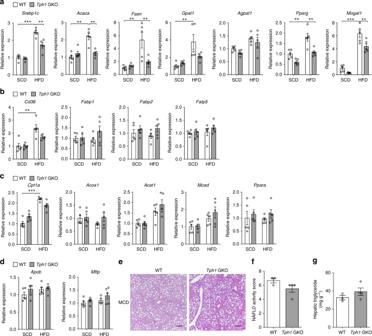Fig. 3 Gut-derived 5-HT regulates lipogenic pathways in the liver.a–dThe 12-week-old WT andTph1GKO mice were fed SCD or HFD for 8 weeks. Relative mRNA expression of genes involved in lipogenesis (a), FA uptake (b), FA oxidation (c), and VLDL secretion (d) as assessed by qRT-PCR in liver;n= 5 per group.e–gThe 8-week-old WT andTph1GKO mice were fed MCD diet for 6 weeks.eRepresentative liver histology by H&E staining. Scale bars, 100 μm.fNAS;n= 3–4 per group.gHepatic triglyceride levels;n= 3–4 per group. Data are expressed as the means ± SEM. **P< 0.01, ***P< 0.001, Student’st-test (f,g) or one-way ANOVA with post hoc Tukey’s test (a–d) 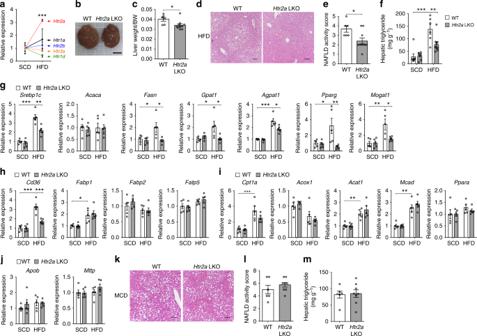Fig. 4 HTR2A mediates the lipogenic action of GDS in the liver.aRelative mRNA expression of indicated HTRs as assessed by qRT-PCR in liver of SCD- and HFD-fed C57BL/6J mice;n= 4 per group.b–jThe 12-week-old WT andHtr2aLKO mice were fed SCD or HFD for 8 weeks. Representative gross liver image (b) and liver weight (c) of HFD-fed WT andHtr2aLKO mice;n= 6–10 per group. Scale bar, 1 cm (b).dRepresentative liver histology by H&E staining from HFD-fed WT andHtr2aLKO mice. Scale bars, 100 μm.eNAS of HFD-fed WT andHtr2aLKO mice;n= 6–10 per group.fHepatic triglyceride levels;n= 6–10 per group.g–jRelative mRNA expression of genes involved in lipogenesis (g), FA uptake (h), FA oxidation (i), and VLDL secretion (j) as assessed by qRT-PCR in liver;n= 5 per group.k–mThe 8-week-old WT andHtr2aLKO mice were fed MCD diet for 6 weeks.kRepresentative liver histology by H&E staining. Scale bars, 100 μm.lNAS;n= 6–8 per group.mHepatic triglyceride levels;n= 6–8 per group. Data are expressed as the means ± SEM. *P< 0.5, **P< 0.01, ***P< 0.001, Student’st-test (a,c,e,l,m) or one-way ANOVA with post hoc Tukey’s test (f–j) 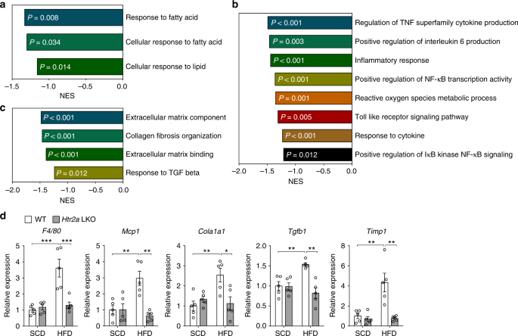Fig. 5 HTR2A mediates the inflammatory and fibrogenic action of GDS in the liver.a–dThe 12-week-old WT andHtr2aLKO mice were fed HFD for 8 weeks.a–cGO gene sets were analyzed by GSEA for HFD-fedHtr2aLKO mice livers compared with WT littermates livers. Gene sets related to hepatic steatosis (a), inflammation (b), and fibrosis (c);n= 3 per group.dRelative mRNA expression of genes involved in inflammation and fibrosis as assessed by qRT-PCR in liver;n= 5 per group. Data are expressed as the means ± SEM. *P< 0.5, **P< 0.01, ***P< 0.001, one-way ANOVA with post hoc Tukey’s test (d) 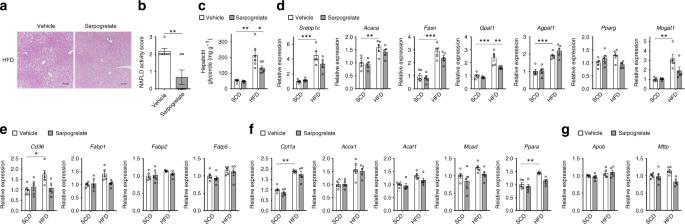Fig. 6 HTR2A antagonist ameliorates HFD-induced hepatic steatosis.a–gThe 12-week-old mice were fed SCD or HFD for 8 weeks and were treated with vehicle or sarpogrelate daily per os.aRepresentative liver histology by H&E staining from HFD-fed vehicle and sarpogrelate treated mice. Scale bars, 100 μm.bNAS of HFD-fed vehicle and sarpogrelate-treated mice;n= 6 per group.cHepatic triglyceride levels;n= 5–6 per group.d–gRelative mRNA expression of genes involved in lipogenesis (d), FA uptake (e), FA oxidation (f), and VLDL secretion (g) as assessed by qRT-PCR in liver;n= 5 per group. Data are expressed as the means ± SEM. *P< 0.5, **P< 0.01, ***P< 0.001, Student’st-test (b) or one-way ANOVA with post hoc Tukey’s test (c–g) The levels of significance indicated in the graphs are * P < 0.05, ** P < 0.01, and *** P < 0.001. Reporting Summary Further information on research design is available in the Nature Research Reporting Summary linked to this article.